S-nitrosothiols regulate nitric oxide production and storage in plants through the nitrogen assimilation pathway Nitrogen assimilation plays a vital role in plant metabolism. Assimilation of nitrate, the primary source of nitrogen in soil, is linked to the generation of the redox signal nitric oxide (NO). An important mechanism by which NO regulates plant development and stress responses is through S -nitrosylation, that is, covalent attachment of NO to cysteine residues to form S -nitrosothiols (SNO). Despite the importance of nitrogen assimilation and NO signalling, it remains largely unknown how these pathways are interconnected. Here we show that SNO signalling suppresses both nitrate uptake and reduction by transporters and reductases, respectively, to fine tune nitrate homeostasis. Moreover, NO derived from nitrate assimilation suppresses the redox enzyme S -nitrosoglutathione Reductase 1 (GSNOR1) by S -nitrosylation, preventing scavenging of S -nitrosoglutathione, a major cellular bio-reservoir of NO. Hence, our data demonstrates that (S)NO controls its own generation and scavenging by modulating nitrate assimilation and GSNOR1 activity. Nitrogen is a conspicuous building block of many central biomolecules, such as nucleic acids, amino acids and cofactors. The primary source of nitrogen available to land plants is inorganic nitrate (NO 3 − ), the concentration of which can vary from micromolar to millimolar amounts in soils [1] . To cope with such large fluctuations in nitrate availability, higher plants have evolved sophisticated high-affinity and low-affinity transport systems [2] , [3] . These systems rely mainly on two families of membrane-bound nitrate transporters (NRTs) of which NRT2 members are high affinity, while most members of NRT1 are low-affinity NRTs [2] , [3] . NRT2.1 and NRT1.1 (firstly identified as CHL1, for chlorate resistant 1) are particularly important for nitrate uptake by roots of Arabidopsis thaliana plants [4] . AtNRT2.1 is a pure high-affinity NRT that is repressed by high nitrate levels and activated under low nitrate conditions [5] . AtNRT1.1 is an exception in the NRT1 family being a dual-affinity NRT: it normally has low-affinity uptake but can change to the high-affinity mode under low nitrate levels [6] , [7] . The switch from low- to high-affinity transport is mediated by phosphorylation at Thr101 residue of NRT1.1, which enhances its affinity to nitrate [8] , [9] , as well as by transcriptional downregulation of NRT1.1 and upregulation of NRT2.1 allowing scavenging of available nitrate [2] , [7] . Once taken up by roots, nitrate is mainly transported to shoots for further assimilation and in leaves it is reduced to nitrite (NO 2 − ) by the activity of NAD(P)H-dependent cytosolic nitrate reductases (NR). Nitrite, in turn, is promptly removed from cells or transported to chloroplasts where it is reduced by nitrite reductase into ammonium (NH 4 + ) for further assimilation into organic compounds by the glutamine synthetase/glutamine-2-oxoglutarate aminotransferase system [1] , [10] , [11] . In Arabidopsis , the catalytic activity of NR, which is considered limiting to nitrogen assimilatory pathways [12] , [13] , is conferred by the genes NIA1 and NIA2 . Double mutant nia1 nia2 plants display poor growth on media with nitrate as the sole nitrogen source, which is in part due to the lack of nitrogen incorporation into amino acids [14] . Curiously, gene expression of NRT1.1 and NRT2.1 transporters is constitutively upregulated in roots of nia1 nia2 plants, suggesting that NR activity or a nitrogen-containing metabolite derived from nitrate reduction feedback regulate uptake systems [15] . However, the identity of this regulatory metabolite remains obscure [15] , [16] . In addition to its reduction to NH 4 + , nitrite can be reduced to nitric oxide (NO) via non-enzymatic as well as various enzymatic pathways [17] , [18] . High levels of nitrite allow NR to reduce this assimilate into NO [19] , [20] , although genetic evidence suggests that the main role of NR in NO biosynthesis is the production of nitrite [21] , [22] . L -arginine, polyamines and hydroxylamines are also potential sources for NO synthesis in higher plants; however, the molecular mechanisms responsible for these activities have not been identified so far [17] , [18] , [23] . NO is a free radical with a wide range of important signalling functions in all eukaryotes. Accordingly, Arabidopsis NO-overproducing nox1 (also known as cue1-6 ) mutants accumulate elevated levels of NO and exhibit defects in floral transition, root apical meristems and pathogen-induced programmed cell death [24] , [25] , [26] . The underlying mechanisms of NO action rely on its physicochemical properties that allow reactivity with different kinds of biomolecules, thereby altering the redox state of their active groups. NO and its derivatives can react with thiols, tyrosine residues, metal centres and reactive oxygen species [17] , [27] . Particularly, addition of NO to cysteine thiols results in the formation of S -nitrosothiols (SNO), which have been shown to alter the activity, localization or conformation of target proteins [27] , [28] . NO may also react with glutathione (GSH) to form S- nitrosoglutathione (GSNO), which is thought to be a major cellular reservoir of NO capable of generating protein-SNO. Cellular GSNO levels are controlled by the evolutionary conserved, cytosolic enzyme GSNO reductase 1 (GSNOR1), which catalyses the NADH-dependent reduction of GSNO to oxidized GSH and ammonium [29] , [30] , [31] . Arabidopsis plants with impaired GSNOR1 function display elevated levels of protein-SNO and exhibit deficiencies in development, immunity and thermotolerance, indicating that GSNOR1 indirectly controls the level of biologically active protein-SNO [31] , [32] , [33] , [34] , [35] , [36] . Taken together, these studies clearly indicate that the generation and scavenging of NO is connected to molecular pathways of nitrogen assimilation. However, it remains unclear if nitrate or other nitrate-derived metabolites directly affect NO signalling, and vice versa, if NO signalling influences nitrogen homeostasis [37] . Here we provide genetic and biochemical evidence for intimate interplay between nitrate assimilation and NO signalling. We identified novel NO-mediated feedback pathways that regulate the transcription of NRTs and enzymatic activities of NR as well as GSNOR1 by redox-based post-translational modification. Our data reveal that nitrate assimilation and NO signalling are connected in unexpected ways, allowing plants to fine tune NO generation and scavenging. NO signalling feedback regulates nitrogen assimilation Because significant amounts of NO and derived SNO result from the nitrogen assimilation pathway, we considered that NO may feedback regulate this pathway. Nitrogen assimilation commences by the uptake of nitrate by low- and high-affinity transport systems, in which the NRT1.1 and NRT2.1 transporter genes play key roles [2] , [3] . We assessed the expression of these genes in roots of wild-type (WT) plants as well as the NO and SNO signalling mutants, nox1 (ref. 24 ) and gsnor1 (ref. 34 ) (also known as par2-1 ). While nox1 plants overproduce free NO, gsnor1 plants accumulate high levels of GSNO [28] , a more stable redox form of NO. Compared with WT plants grown under moderate nitrate availability, the expression of NRT2.1 was strongly suppressed in both nox1 and gsnor1 mutants, whereas the expression of NRT1.1 remained unchanged ( Fig. 1a ). Accordingly, exogenous treatment of WT plants with GSNO or the alternative NO donor, DEA/NO, also led to the inhibition of NRT2.1 expression but left NRT1.1 expression unaltered ( Fig. 1b ). These findings suggest that elevated NO and SNO levels induce a switch from high- to low-affinity nitrate transport. 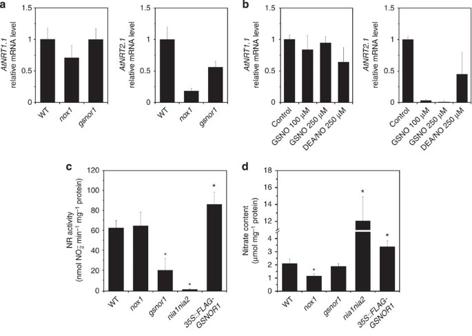Figure 1: Nitrate uptake and reduction in plants with altered NO signalling. (a) Expression of the NRT marker genesNRT1.1andNRT2.1in the roots of WT,nox1andgsnor1plants was determined by quantitative reverse transcriptase-PCR (qRT–PCR) and normalized to expression ofACT2.Error bars represent s.d. (n=3). (b) Effect of GSNO on nitrate-induced expression ofNRTgenes in roots. WT seedlings grown in half-strength MS medium (9.4 mM KNO3and 10.3 mM NH4NO3) were incubated for 3 h in water with 1 mM nitrate (KNO3), in the absence or presence of GSNO or DEA/NO.NRTexpression was determined by qRT–PCR and normalized to expression ofACT2.Error bars represent s.d. (n=3). (c) NR activity and (d) nitrate (NO3−) content determined in leaf extracts of WT plants and genotypes with enhanced (nox1andgsnor1) or impaired (nia1 nia2and35S::FLAG-GSNOR1) (S)NO homeostasis, after 6 hours of light. Data points represent means±s.d. of three independent experiments. Asterisks indicate statistical differences from the WT (Student’st-test,P<0.05). Figure 1: Nitrate uptake and reduction in plants with altered NO signalling. ( a ) Expression of the NRT marker genes NRT1.1 and NRT2.1 in the roots of WT, nox1 and gsnor1 plants was determined by quantitative reverse transcriptase-PCR (qRT–PCR) and normalized to expression of ACT2. Error bars represent s.d. ( n =3). ( b ) Effect of GSNO on nitrate-induced expression of NRT genes in roots. WT seedlings grown in half-strength MS medium (9.4 mM KNO 3 and 10.3 mM NH 4 NO 3 ) were incubated for 3 h in water with 1 mM nitrate (KNO 3 ), in the absence or presence of GSNO or DEA/NO. NRT expression was determined by qRT–PCR and normalized to expression of ACT2. Error bars represent s.d. ( n =3). ( c ) NR activity and ( d ) nitrate (NO 3 − ) content determined in leaf extracts of WT plants and genotypes with enhanced ( nox1 and gsnor1 ) or impaired ( nia1 nia2 and 35S::FLAG-GSNOR1 ) (S)NO homeostasis, after 6 hours of light. Data points represent means±s.d. of three independent experiments. Asterisks indicate statistical differences from the WT (Student’s t -test, P <0.05). Full size image Once taken up into the root, nitrate is mainly transported to the shoots where it is assimilated at the expense of photosynthetic reducing power [2] . In leaves, nitrate is reduced to nitrite by the cytosolic enzyme NR. To examine if NO also regulates this rate-limiting step in nitrogen assimilation, we measured NR activity in leaves of the genotypes with altered (S)NO homeostasis ( Fig. 1c ). Compared with WT, gsnor1 mutant plants exhibited strongly reduced NR activity, while GSNOR1 -overexpressing plants ( 35S::FLAG-GSNOR1 , Supplementary Fig. 1a,b ) displayed enhanced NR activity. Surprisingly, however, mutant nox1 plants, which only accumulate 30–40% more SNO than WT plants under basal conditions [26] , did not exhibit altered NR activity ( Fig. 1c ). Together with the fact that expression of the NR gene NIA2 was indifferent in all mutants ( Supplementary Fig. 1c,d ), these data suggest that GSNO and free NO differentially affect NR activity. To understand the cumulative consequences of (S)NO-modulated nitrate transport and reduction, we also measured nitrate contents of mutant leaves and compared them with WT and NR double mutant nia1 nia2 leaves, the latter of which is known to accumulate high levels of nitrate due to lack of NR activity [15] . Figure 1d shows that nox1 plants accumulated significantly less nitrate than the WT, likely caused by partial switching to the low-affinity transport system in these mutants ( Fig. 1a ). However, in gsnor1 plants, activation of the low-affinity transport system in conjunction with reduced NR activity apparently resulted in relatively normal nitrate levels. Instead, a regulatory role for GSNO only became apparent in 35S::FLAG-GSNOR1 plants, which accumulated elevated levels of nitrate ( Fig. 1d ). Taken together, these findings indicate that NO and SNO modulate nitrogen assimilation by differentially inhibiting nitrate uptake and reduction. To assess the biological impact of (S)NO on nitrate assimilation, we analysed the vigour of (S)NO signalling mutants by measuring growth and biomass accumulation parameters ( Fig. 2a–d ). As expected, the inability of nia1 nia2 plants to reduce nitrate led to reduced leaf area and a decrease in dry shoot weight compared with WT. Like nia1 nia2 , mutant nox1 and gsnor1 plants also displayed strongly decreased growth vigour. Conversely, leaf area and biomass growth tended to increase, albeit not always statistically significant, in GSNOR1-overexpressing 35S::FLAG-GSNOR1 plants ( Fig. 2a–d ). These findings suggest that (S)NO-mediated suppression of nitrate assimilation may have dramatic effects on plant growth. To confirm the poor growth vigour phenotypes of (S)NO mutants were due to decreased nitrate assimilation, we sought to bypass this pathway by the exogenous addition of glutamine (Gln), the main end product of nitrate assimilation. Addition of Gln to WT plants did not further improve growth compared with nitrate-replete conditions ( Supplementary Fig. 2 ). Importantly, however, irrigation of nox1 and gsnor1 mutants in the presence of Gln recovered growth vigour of gsnor1 , but not that of nox1 , to levels comparable to those of WT and 35S::FLAG-GSNOR1 plants ( Fig. 2a–d ). Thus, bypassing both nitrate uptake and reduction by feeding Gln rescued the gsnor1 phenotype, while suppression of N assimilation may not be the only cause for lack of growth vigour in nox1 plants. In contrast to GSNOR1 that is directly involved in NO homeostasis, the metabolic changes in nox1 that lead to an increase in NO production are indirect. The nox1 mutant is defective in a phosphoenolpyruvate/phosphate translocator that imports phosphoenolpyruvate for the synthesis of aromatic amino acids and related compounds through the shikimate pathway [38] . Consequently, nox1 mutants display an overall marked increase in the levels of free amino acids, including L -arginine, a precursor of NO [24] ( Supplementary Fig. 3 ). In addition, this mutant exhibits an imbalance of aromatic versus non-aromatic amino acids and a marked reduction in secondary phenolic compounds that are dependent on the shikimate pathway for precursors, severely compromising the establishment of photoautotrophic growth [38] . Thus, alterations of amino acid levels as a direct consequence of the nox1 mutation are not expected to be complemented by simply adding Gln, as other imbalances are not corrected by this treatment. Accordingly, the effect of the nox1 mutation on biomass is much more severe than the nia1 nia2 knockout mutation ( Fig. 2a–d ), indicating that mechanisms unrelated to nitrate assimilation underpin the nox1 phenotype. In contrast, our data indicate that mutation of GSNOR1 affected plant growth by inhibiting nitrate uptake and assimilation ( Fig. 1 ), and accordingly, this phenotype can be rescued by addition of Gln ( Fig. 2a–d ). 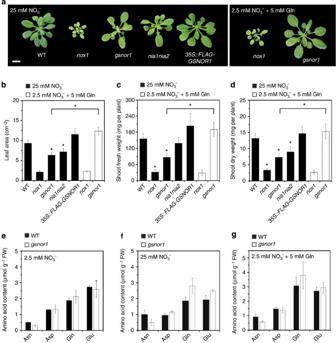Figure 2: Growth vigour and amino acid content of genotypes with impaired and enhanced (S)NO signalling. (a) Phenotype, (b) leaf area, (c) shoot fresh weight and (d) shoot dry weight of 4-week-old plants grown on perlite:vermiculite (1:1) under 12 h/12 h light/dark and irrigated three times a week with a MS nutrient solution containing 25 mM nitrate (half KNO3and half NH4NO3) (black bars) or with 2.5 mM nitrate and 5 mM glutamine (white bars). Scale bar, 1 cm. Data points represent means±s.d. (n=15 plants). (e–g) Contents of primary transported amino acids in WT andgsnor1leaves. Asn, asparagine; Asp, aspartate; Gln, glutamine; Glu, glutamate. Data represent means±s.d. of three independent analyses. Asterisks indicate statistically significant differences from WT (Student’st-test,P<0.05). Figure 2: Growth vigour and amino acid content of genotypes with impaired and enhanced (S)NO signalling. ( a ) Phenotype, ( b ) leaf area, ( c ) shoot fresh weight and ( d ) shoot dry weight of 4-week-old plants grown on perlite:vermiculite (1:1) under 12 h/12 h light/dark and irrigated three times a week with a MS nutrient solution containing 25 mM nitrate (half KNO 3 and half NH 4 NO 3 ) (black bars) or with 2.5 mM nitrate and 5 mM glutamine (white bars). Scale bar, 1 cm. Data points represent means±s.d. ( n =15 plants). ( e – g ) Contents of primary transported amino acids in WT and gsnor1 leaves. Asn, asparagine; Asp, aspartate; Gln, glutamine; Glu, glutamate. Data represent means±s.d. of three independent analyses. Asterisks indicate statistically significant differences from WT (Student’s t -test, P <0.05). Full size image To further establish that suppressed nitrate assimilation underpins the poor primary productivity phenotype of gsnor1 plants, we assessed the global accumulation of amino acids in this mutant ( Supplementary Fig. 3 ). Particularly the accumulation of glutamine (Gln), glutamate (Glu), asparagine (Asn), and aspartate (Asp) are informative for nitrogen homeostasis, because they represent the primary transported amino acids derived from ammonium [11] . Several observations made in gsnor1 mutants support the notion that (S)NO-mediated suppression of nitrate assimilation affects primary productivity. First, low nitrogen conditions stimulate the formation of Gln and Glu because of their comparatively lower nitrogen-to-carbon ratios (2N:5C for Gln and 1N:5C for Glu). Importantly, even in the presence of high nitrate, gsnor1 plants accumulated more Gln and Glu compared with the WT ( Fig. 2e,f ), indicating that these mutants were suffering from nitrogen shortage. Second, compared with Gln and Glu, the amino acid Asn is rich in nitrogen (2N:4C ratio) and its production is therefore avoided under low nitrogen availability. Despite the presence of 25 mM nitrate, mutant gsnor1 plants contained decreased levels of Asn compared with WT ( Fig. 2e,f ), further indicating that these mutants experience a shortage in nitrogen. Finally, in both WT and gsnor1 plants, exogenous addition of 5 mM Gln led to an expected rise in endogenous Gln and also increased Asn content, while the levels of Glu and Asp remained largely unchanged compared with the low nitrate regime ( Fig. 2e–g , Supplementary Fig. 3 ). Taken together, these data indicate that (S)NO are important regulators of nitrate assimilation and thus, plant growth and development. Nitrogen metabolism regulates GSNOR1 activity Given the impact of GSNOR1 on nitrate assimilation, we considered that GSNOR1 activity may be feedback regulated by nitrate. To examine this possibility, we grew WT plants under high nitrate availabilities that caused good growth vigour (25 and 40 mM), as well as lower nitrate availabilities (1 and 2.5 mM) that resulted in poor biomass accumulation ( Supplementary Fig. 2 ). Because the irrigated nutrient solution was not compensated with any other nitrogen source, nitrate concentrations lower than 2.5 mM appeared undesirably detrimental for plant growth and development. Therefore we selected 2.5 and 25 mM nitrate concentrations for further experimentation. In addition, as the nitrate concentration of nutrient solutions was composed of half KNO 3 and half NH 4 NO 3 , we checked the possibility that the effects observed could partially be attributed to NH 4 + . However, when the concentration of NH 4 + in the nutrient solution was reduced by 10 times (from 12.5–1.25 mM), parameters of biomass growth of WT plants were comparable ( Supplementary Fig. 4 ), indicating that the effect of ammonium in determining plant growth vigour was negligible under our conditions. Interestingly, increasing nitrate availability from 2.5 to 25 mM reduced mean GSNOR1 activity by 35%±8% while significantly enhancing NR activity ( Fig. 3a,b ). Additional increase in nitrate availability to 40 mM did not suppress GSNOR activity any further, while intermediate nitrate levels (12.5 mM) reduced GSNOR activity by ~10% ( Supplementary Fig. 5 ). These data suggest that nitrate levels may regulate GSNOR1 activity. However, mutant nia1 nia2 plants that are void of NR activity ( Figs 1c and 3b ) and accumulate elevated levels of endogenous nitrate [15] ( Fig. 1d ), did not exhibit reduced but rather slightly elevated GSNOR1 activity ( Fig. 3a ). Thus, instead of nitrate, a metabolite downstream of NR-catalysed nitrate reduction may be responsible for inhibition of GSNOR1 activity. 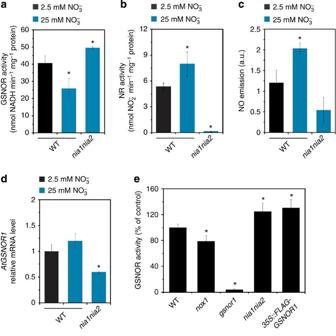Figure 3: Nitrate-derived NO suppresses activity of GSNOR1. (a) GSNOR activity, (b) NR activity, (c) NO emission and (d)GSNOR1gene expression measured in leaf extracts of WT andnia1 nia2plants grown under low or high nitrate availability. Plants were grown in perlite:vermiculite (1:1) under a 12/12 h light/dark period and irrigated three times a week with MS nutrient solution containing 2.5 or 25 mM nitrate (half KNO3and half NH4NO3). All measurements were taken 6 hours post light exposure. Relative expression ofGSNOR1in (d) was determined by quantitative reverse transcriptase-PCR and normalized to expression ofACT2. (e) GSNOR activity in genotypes with impaired and enhanced (S) NO signalling. Plants were grown in soil with a photoperiod of 16/8 h light/dark and irrigated with water as needed. Data points represent means±s.d. of three independent experiments. Asterisks indicate significant differences from the WT (Student’st-test,P<0.05). Figure 3: Nitrate-derived NO suppresses activity of GSNOR1. ( a ) GSNOR activity, ( b ) NR activity, ( c ) NO emission and ( d ) GSNOR1 gene expression measured in leaf extracts of WT and nia1 nia2 plants grown under low or high nitrate availability. Plants were grown in perlite:vermiculite (1:1) under a 12/12 h light/dark period and irrigated three times a week with MS nutrient solution containing 2.5 or 25 mM nitrate (half KNO 3 and half NH 4 NO 3 ). All measurements were taken 6 hours post light exposure. Relative expression of GSNOR1 in ( d ) was determined by quantitative reverse transcriptase-PCR and normalized to expression of ACT2 . ( e ) GSNOR activity in genotypes with impaired and enhanced (S) NO signalling. Plants were grown in soil with a photoperiod of 16/8 h light/dark and irrigated with water as needed. Data points represent means±s.d. of three independent experiments. Asterisks indicate significant differences from the WT (Student’s t -test, P <0.05). Full size image Nitrite is the first reductive metabolite downstream of nitrate and in elevated concentrations can be converted into NO [21] , [22] , [39] . Therefore, we measured NO emission in plants grown under low and high nitrate availability. High concentrations of nitrate promoted NO emission in WT plants ( Fig. 3c and Supplementary Fig. 6 ). Despite having elevated endogenous nitrate levels, nia1 nia2 plants did not show elevated NO emission when grown under higher nitrate, indicating that high nitrate availability leads to NR-mediated generation of NO. Because nitrate-induced, NR-mediated NO production was associated with reduced enzymatic activity of GSNOR1 ( Fig. 3a–c ) but not gene expression ( Fig. 3d ), we considered a more direct role for NO in regulating the GSNOR1 enzyme. We examined this in genotypes with impaired and enhanced (S)NO signalling. Importantly, NO-overproducing nox1 mutants displayed significantly reduced GSNOR1 activity ( Fig. 3e ). Conversely, nia1 nia2 double mutants that cannot synthesize NO through the NR pathway, exhibited increased GSNOR1 activity to similar levels as 35S::FLAG-GSNOR1 plants. Collectively, these data suggest that the nitrogen assimilatory pathway inhibits GSNOR1 by a post-transcriptional, NO-dependent mechanism. NO-induced S -nitrosylation inhibits GSNOR1 To further investigate if GSNOR1 is inhibited directly by NO or by other nitrogen assimilates, we measured its in vitro activity in pharmacological assays. Addition of the redox-active NO donors diethylamine NONOate (DEA/NO) and Cys-NO to WT leaf extracts resulted in dose-dependent inhibition of GSNOR1 with 15–30% decrease in activity already at only 50 μM of NO donors and over 60% at 250 μM ( Fig. 4a ). In contrast, the redox-active molecules, GSH and L -Cysteine that do not donate NO, had relatively little effect on GSNOR1 activity. Similarly, incubation with physiologically relevant concentrations of nitrogen assimilates (nitrate, nitrite and ammonium) did not affect GSNOR1 activity with the exception of high concentrations of the NO-related signal molecule peroxynitrite (ONOO − ), which is formed by the reaction of NO and O 2 − ( Fig. 4b ) [40] . Furthermore, when WT plants were fumigated for 12 h with 60 p.p.m. of NO gas, GSNOR activity in leaves was nearly 40% lower when compared with those exposed to normal air (44.6±2.6 versus 71.7±5.4 nmol NADH min −1 per mg protein) ( Fig. 4c ). Taken together, these data demonstrate a direct inhibitory effect of NO on GSNOR activity. 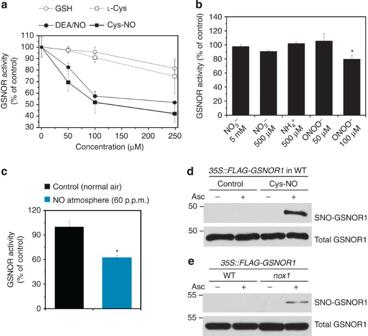Figure 4: NO inhibits GSNOR1 byS-nitrosylation. (a) Dose response of GSNOR activity in WT leaf extracts supplemented with theS-nitrosylating agents DEA/NO and Cys-NO or the redox-active molecules GSH andL-Cys. (b) GSNOR activity in WT leaf extracts supplemented with indicated intermediates of the nitrogen assimilation pathway. (c) GSNOR activity in leaf extracts of WT plants fumigated with NO gas (60 p.p.m.) or with normal air for 12 h. (d) Cys-NO inducedS-nitrosylation of GSNOR1in vitro. Leaf extracts from35S::FLAG-GSNOR1plants in WT background were exposed to Cys-NO and subjected to the biotin switch technique. Total GSNOR1 protein ensures equal protein loading. The position of a 50-kDa marker is indicated. (e)In vivo S-nitrosylation of GSNOR1 using a35S::FLAG-GSNOR1construct in WT andnox1background. SNO-GSNOR1 was analysed and detected as ind. The position of a 55-kDa marker is indicated. Data points fromatocrepresent means±s.d. of at least three independent experiments. Asterisks indicate significant differences from the controls (Student’st-test,P<0.05). Figure 4: NO inhibits GSNOR1 by S -nitrosylation. ( a ) Dose response of GSNOR activity in WT leaf extracts supplemented with the S- nitrosylating agents DEA/NO and Cys-NO or the redox-active molecules GSH and L -Cys. ( b ) GSNOR activity in WT leaf extracts supplemented with indicated intermediates of the nitrogen assimilation pathway. ( c ) GSNOR activity in leaf extracts of WT plants fumigated with NO gas (60 p.p.m.) or with normal air for 12 h. ( d ) Cys-NO induced S -nitrosylation of GSNOR1 in vitro . Leaf extracts from 35S::FLAG-GSNOR1 plants in WT background were exposed to Cys-NO and subjected to the biotin switch technique. Total GSNOR1 protein ensures equal protein loading. The position of a 50-kDa marker is indicated. ( e ) In vivo S -nitrosylation of GSNOR1 using a 35S::FLAG-GSNOR1 construct in WT and nox1 background. SNO-GSNOR1 was analysed and detected as in d . The position of a 55-kDa marker is indicated. Data points from a to c represent means±s.d. of at least three independent experiments. Asterisks indicate significant differences from the controls (Student’s t -test, P <0.05). Full size image NO has been well documented to regulate protein function by S -nitrosylation [24] , [41] . Therefore, we employed the biotin switch technique to examine if GNSOR1 is subjected to S -nitrosylation. This technique relies on specific reduction of SNO groups by ascorbate followed by their labelling with biotin [42] . Extracts of plants expressing 35S::FLAG-GSNOR1 ( Supplementary Figs 1 and 7 ) were treated with or without the NO donor Cys-NO and subjected to the biotin switch technique. Figure 4d shows that Cys-NO induced strong S -nitrosylation of FLAG-GSNOR1 protein that was completely dependent on addition of ascorbate during biotin switching, indicating that GSNOR1 can be S -nitrosylated in vitro . Next, we assessed if GSNOR1 is also S -nitrosylated in vivo by examining SNO modifications in NO-overproducing nox1 plants that exhibit reduced GSNOR1 activity ( Fig. 3e ). To that end, we crossed 35S::FLAG-GSNOR1 -expressing plants with nox1 mutants and applied the biotin switch technique on the resulting homozygous progeny in which FLAG-GSNOR1 protein accumulated to comparable levels as the parent line ( Supplementary Fig. 7 ). Whereas most of the FLAG-GSNOR1 protein was unmodified in WT plants, it was significantly S -nitrosylated in nox1 mutants ( Fig. 4e ). Taken together, these data indicate that nitrate-derived NO prevents scavenging of its major storage form by inhibitory S -nitrosylation of GSNOR1. As immobile organisms, plants have evolved to cope with environmental fluctuations by fine tuning metabolic pathways. Nitrogen metabolism is of particular importance as its intermediates influence plant development and responses to stress. Our study shows that NO, one of the end products of nitrogen metabolism, feedback regulates flux through nitrate assimilation pathways and controls its bioavailability by modulating its own consumption as depicted in Fig. 5 . 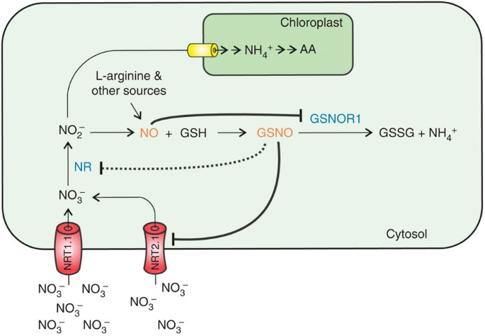Figure 5: Schematic model for the control of nitrogen assimilation in plants through NO signalling. Nitrate (NO3−) is taken up by NRT in roots and reduced in leaves to nitrite (NO2−) by NR. Besides the transport to chloroplasts where it is reduced to ammonium (NH4+) and incorporated into amino acids (AA), nitrite can be reduced to NO by any favourable reducing power. NO is also thought to be generated from other sources, such asL-arginine. NO reacts with reduced glutathione (GSH) producingS-nitrosoglutathione (GSNO), the major cellular reservoir of NO. The levels of GSNO are controlled by the enzyme GSNO reductase (GSNOR1), which catalyses the reduction of GSNO to oxidized glutathione (GSSG) and ammonium (NH3). GSNO inhibits nitrate uptake and reduction and NOS-nitrosylates and inhibits GSNOR1 preventing GSNO degradation. In this way NO, one of the end products of nitrogen metabolism, feedback regulates flux through nitrate assimilation pathway and controls its bioavailability by modulating its own consumption. Figure 5: Schematic model for the control of nitrogen assimilation in plants through NO signalling. Nitrate (NO 3 − ) is taken up by NRT in roots and reduced in leaves to nitrite (NO 2 − ) by NR. Besides the transport to chloroplasts where it is reduced to ammonium (NH 4 + ) and incorporated into amino acids (AA), nitrite can be reduced to NO by any favourable reducing power. NO is also thought to be generated from other sources, such as L -arginine. NO reacts with reduced glutathione (GSH) producing S -nitrosoglutathione (GSNO), the major cellular reservoir of NO. The levels of GSNO are controlled by the enzyme GSNO reductase (GSNOR1), which catalyses the reduction of GSNO to oxidized glutathione (GSSG) and ammonium (NH 3 ). GSNO inhibits nitrate uptake and reduction and NO S -nitrosylates and inhibits GSNOR1 preventing GSNO degradation. In this way NO, one of the end products of nitrogen metabolism, feedback regulates flux through nitrate assimilation pathway and controls its bioavailability by modulating its own consumption. Full size image Previously it has been suggested that a metabolite resulting from nitrate reduction may feedback regulate nitrate uptake systems, but the identity of this metabolite remained unknown [15] , [16] , [23] . Genetic manipulation of NO signalling in our experiments illustrated that NO controls flux through nitrogen assimilatory pathway by modulating the expression of NRTs and activity of NR ( Fig. 1 ). Mutants that accumulate NO or GSNO displayed a classical switch in gene expression from high- to low-affinity transport, which is typically associated with decreased uptake of exogenous nitrate [4] . Moreover, genetically elevated levels of GSNO inhibited the activity of NR, while reduced levels promoted its activity. We show that the cumulative effects of perturbed NO signalling on nitrate uptake and reduction determined leaf nitrate content ( Fig. 1 ), homeostasis of primary transport amino acids ( Fig. 2e–g and Supplementary Fig. 3 ) and affected plant growth vigour ( Fig. 2a–d ). This NO-dependent mechanism may ensure the adjustment of plant growth according to nitrate availability. In higher plants, NO is probably generated through a variety of mechanisms, including NO synthase-like activities, polyamine biosynthetic pathways and mitochondrial or peroxisomal pathways [20] , [23] . Notably, however, significant amounts of NO are also thought to be generated through a NR-dependent process, which may be particularly important in root architecture [43] , floral transition [44] , responses to abiotic stresses [45] , [46] and immune responses [22] , [47] . Thus, by suppressing nitrate uptake and reduction, NO may not only regulate nitrogen assimilation fluxes, it probably also feedback regulates its own generation. Remarkably, NR activity was coupled to the level of functional GSNOR1 ( Figs 1c and 3e ). As GSNO often regulates enzyme activity through S -nitrosylation, it is tempting to speculate that NR is also subject to this post-translational modification. Indeed, NR is known to be regulated by other post-translational mechanisms, including phosphorylation and degradation. NIA2 was shown to interact with mitogen-activated protein kinase 6, resulting in site-specific phosphorylation that promoted NR activity [43] . Furthermore, phosphorylation of a distinct residue was shown to recruit inhibitory 14-3-3 proteins and may also promote NR proteolysis [48] , [49] , [50] . While we observed impaired NR activity in gsnor1 plants that are deficient in functional GSNOR1, no effect was seen in NO-overproducing nox1 plants ( Fig. 1 ). Because NO donor stereochemistry and structure as well as allosteric effectors have a large influence on SNO reactivity [51] , these data imply that NO and GSNO do not always modify the same target proteins. Indeed, NO radicals are thought to S -nitrosylate proteins directly through a radical-mediated pathway or indirectly via higher oxides of NO, whereas GSNO trans -nitrosylates cysteine residues [52] . Feeding experiments not only confirmed the previously described ability of nitrate to promote NR activity [53] , they also demonstrated that elevated nitrate levels suppress GSNOR1 activity ( Fig. 3 ). GSNOR1 plays an important role in controlling the cellular levels of GSNO, which is thought to be the main NO reservoir in cells. Accordingly, the mutation of GSNOR1 leads to elevated levels of protein SNO [31] , indicating that GSNO functions as a potent cellular NO donor. As high NR activity promoted generation of NO ( Fig. 3b,c ), inhibition of GSNOR1 may be necessary to amplify SNO signals. Indeed, storing NO as GSNO dramatically prolongs its half-life [54] , perhaps enabling plants to utilize NO more efficiently while curbing loss due to emission. Taken together, our data illustrate that nitrate availability promotes formation of a more stable pool of NO, which in turn feedback regulates nitrate assimilation, allowing plants to finely tune nitrogen homeostasis. They also indicate that nitrogen-based nutrient availability may influence a variety of NO-mediated signalling events. This is supported by recent reports showing that the form of nitrogen assimilation determines NO-mediated immune responses [55] , [56] . Arabidopsis nia1 nia2 mutants are susceptible to the bacterial pathogen Pseudomonas syringae , even after amino acid recovery by feeding with Gln [56] . Furthermore, treatment of WT tobacco plants with ammonium bypassed NR-mediated generation of NO and consequently compromised immune responses [55] . In contrast, application of nitrate or nitrite promoted both NO formation and immune-induced hypersensitive cell death, a process that restricts pathogen growth and is known to be stimulated by SNO [26] , [55] , [56] . It should be noted that although nitrate-induced NO emission was strongly reduced in absence of functional NR, residual NR-independent NO emission is still observed in nia1 nia2 ( Fig. 3c , Supplementary Fig. 6 ). Taken together with the fact that NR-independent NO overproduction in nox1 mutants decreased nitrate content in part by suppressing nitrate transport ( Fig. 1 ), these data indicate that NR-independent NO production may also contribute to nitrate homeostasis ( Fig. 5 ). We showed that in vitro application of intermediates of nitrate assimilation did not affect GSNOR1 activity, whereas application of NO donors specifically blocked its activity even at low dosage ( Fig. 4a,b ). Accordingly, genetic manipulation of NO levels in nox1 and nia1 nia2 plants ( Fig. 3e ) and direct fumigation of NO gas on WT plants ( Fig. 4c ) also impacted GSNOR1 activity in planta . Remarkably, the inhibitory effect of NO was associated with S -nitrosylation of GSNOR1 both in vitro and in vivo ( Fig. 4d,e ), indicating that this NO-scavenging enzyme is itself subject to direct regulation by NO. So how does S -nitrosylation inhibit the activity of GSNOR1? Elucidation of the crystal structure of tomato GSNOR1 indicated the presence of a number of important cysteine residues that might serve as sites for S -nitrosylation [57] . Two clusters of cysteine residues coordinate binding of two zinc atoms with catalytic and structural roles. The catalytic zinc atom may be necessary for coordination of the substrate and coenzyme NAD + . Thus, S -nitrosylation of any cysteine residue within the catalytic cluster could prevent coordination of zinc and disrupt the substrate or NAD + binding pockets. Alternatively, S -nitrosylation of cysteines within the structural cluster may prevent GSNOR1 from folding appropriately. The exact site of S -nitrosylation of GSNOR1 and associated inhibitory mechanism remain to be determined. Regardless of these details, our data show NO directly regulates GSNOR1 through post-translational modification and suggest a novel mechanism by which NO controls its own bioavailability ( Fig. 5 ). Taken together with our biochemical and genetic evidence that nitrate assimilation is feedback repressed by NO, we conclude that NO is at the centre of fine tuning nitrogen homeostasis in plants. These findings raise important considerations for the impacts of nitrogen-based fertilizers on redox-mediated traits in agricultural crops. Nitrogen is a major nutrient required for plant growth and development and for this reason insufficient N in soil severely restricts the use of potential agricultural lands. To circumvent this limitation, application of nitrate-based fertilizers has been the most widely used method to increase crop yields. However, the unutilized nitrate in agricultural fields is one of the main sources of environmental N pollution, as well economic losses [58] . Therefore, understanding the physiological basis involved in the adjustment of plant growth in response to nitrate availability is essential for the development of crop plants either adapted to N-limiting conditions or with high efficiency in nitrogen assimilation [59] . The present identification of NO as a key element for adjustment in plant growth according to nitrate availability generates an important basis for future research programs to attain higher yields and promote a reduction in fertilizer-based environmental pollution. Plant materials, growth conditions and treatments Arabidopsis thaliana Columbia-0 WT and the mutants nia1 nia2 (ref. 14 ), gsnor1 ( par2-1 ) [34] and nox1 ( cue1-6 ) [24] , as well as the transgenic lines 35S::FLAG-GSNOR1 in WT and nox1 backgrounds were grown in soil in a controlled environmental chamber at 20–22 °C, 65% relative humidity and a photoperiod of 16/8 h light/dark. The form and content of N in the soil was not determined and the plants were irrigated with water as needed. Where indicated nitrate availability was controlled by growing plants in perlite:vermiculite (1:1) under a 12/12 h light/dark period. Plants were irrigated with Murashige–Skoog (MS) [60] nutrient solution three times a week. In these treatments, the composition of inorganic N was altered from the original one in a way that nitrate supply was composed of half KNO 3 and half NH 4 NO 3 . Four-week-old plants were used for the experiments. For analysis of gene expression in roots, seeds were surface sterilized with 10% bleach for 5 min, washed three times with sterile water and sown aseptically in petri dishes containing half-strength MS medium (in which the N source is composed of 9.4 mM KNO 3 and 10.3 mM NH 4 NO 3 ). Petri dishes were maintained vertically in a photoperiod of 16/8 h light/dark at 20–22 °C. After 15 days, the seedlings were gently lifted from petri dishes using forceps and analysed immediately or incubated in 10 ml of sterile deionized water containing 1 mM KNO 3 supplemented with or without GSNO or DEA/NO at room temperature for 3 h. Roots were then separated from the shoot with the aid of a scalpel and RNA extraction was carried out as described below. Construction of transgenic 35S::FLAG-GSNOR1 plants The full-length GSNOR1 gene was multiplied from cDNA and TOPO cloned into the Gateway compatible pENTR/SD/D-TOPO vector according to the manufacturer’s instructions (Invitrogen, Carlsbad, CA). The resulting pENTR/ GSNOR1 clone was linearized with the restriction enzyme Mlu I to prevent subsequent transformation of the entry vector into E. coli . Using LR clonase (Invitrogen), the GSNOR1 sequence flanked by the entry vector’s att L recombination sites were recombined into the plant transformation vector pEarleyGate 202 (ref. 61 ), which contains an amino-terminal FLAG epitope tag driven by a cauliflower mosaic virus 35S promoter. The resulting pEarleyGate 202/ 35S::FLAG-GSNOR1 vector was transformed into Agrobacterium tumefaciens strain GV3101(pMP90), which was subsequently used to transform WT plants by floral dipping [62] . Transgenic plants were selected on soil by repeated spraying with glufosinate ammonium. A homozygous transgenic line with appropriate transgene expression was isolated by immunoblotting for FLAG and crossed into nox1 mutants. Plant NO fumigation WT plants grown in perlite:vermiculite (1:1), irrigated with MS nutrient solution containing 12.5 mM nitrate and maintained in a growth chamber with a 12 h photoperiod were fumigated with NO gas [63] . Briefly, plants were transferred to an acrylic fumigation chamber for 12 h. Exposure to NO (60 p.p.m.) was performed by bubbling of NO gas with a continuous flow of 90 ml min −1 (200 ppm diluted in N 2 ) plus 210 ml min −1 of commercial air. In the control assays, a total flow of 300 ml min −1 of air was applied. Subsequently, fumigated leaves were collected and prepared for measurement of GSNOR activity. Measurement of GSNO reductase activity GSNO reductase activity in leaf extracts was measured spectrophotometrically as the rate of NADH oxidation in the presence of GSNO [31] . Briefly, total leaf protein was extracted in 20 mM HEPES buffer (pH 8.0), 0.5 mM EDTA and proteinase inhibitors (50 μg ml −1 TPCK; 50 μg ml −1 TLCK; 0.5 mM PMSF). Protein concentrations were measured with a Bio-Rad Protein Assay Kit II (Bio-Rad, Hercules, CA) according to the manufacturer’s instructions and adjusted to either 62.5 μg (for nia1 nia2 , which have very low protein content) or 125 μg (for all remaining genotypes). Protein extracts were incubated in 1 ml of reaction buffer containing 20 mM HEPES buffer (pH 8.0), 350 μM NADH and 350 μM GSNO. GSNO reductase activity was determined by subtracting NADH oxidation in the absence of GSNO from that in the presence of GSNO. All samples were protected from light during the assay and tested for linearity. Where indicated, protein extracts were preincubated for 20 min with intermediates of nitrogen metabolism or NO signalling molecules at the stated concentrations before addition of the reaction buffer. Measurement of NR activity NR activity was measured as the rate of NO 2 − production [64] . Briefly, total leaf protein was extracted in 20 mM HEPES (pH 8.0), 0.5 mM EDTA, 10 μM FAD, 5 μM Na 2 MoO 4 , 6 mM MgCl 2 and proteinase inhibitors (50 μg ml −1 TPCK; 50 μg ml −1 TLCK; 0.5 mM PMSF). A total of 50 μg protein was incubated in 300 μl of extraction buffer supplemented with 10 mM KNO 3 and 1 mM NADH. Nitrite production was determined by adding equal volumes of 1% sulphanilamide and 0.02% N -(1-naphthyl) ethylenediamine dihydrochloride in 1.5 N HCl, and absorbance measured at 540 nm on a spectrophotometer. The obtained values were compared with those of a standard curve constructed using KNO 2 and normalized by protein content. All samples were protected from light during the assay. Determination of nitrate content Nitrate content was determined by nitration of salicylic acid [65] . Briefly, leaves were ground in liquid nitrogen and resuspended in 20 mM HEPES (pH 8.0). After centrifugation at 10,000 g for 10 min at 4 °C, aliquots of 5 μl of supernatant were mixed with 45 μl of 5% (v/v) salicylic acid in sulfuric acid for 20 min. The solution was neutralized by slowly adding 950 μl of NaOH (2 N). Absorbance was determined at 410 nm and the values obtained were compared with those of a standard curve constructed using KNO 3 and normalized by protein content. Measurement of NO emission NO emission by leaves was determined by fluorometric analysis using 4,5-diamino-fluorescein-2 (ref. 66 ). Briefly, leaf samples of WT and nia1 nia2 plants were incubated in the dark with 10 μM 4,5-diamino-fluorescein-2 dissolved in 10 mM phosphate buffer, pH 8.0. After 1 h incubation, fluorescence emission at 515 nm under an excitation at 495 nm was recorded using an F-4500 spectrofluorometer (Hitachi, Tokyo, Japan). As negative control, leaves were incubated in the presence of 200 μM of the NO scavenger 2-(4-carboxyphenyl)-4,4,5,5-tetramethyl imidazoline-1-oxyl-3-oxide and the residual fluorescence subtracted. Analysis of amino acid content Leaf free amino acids were determined by reversed-phase high-performance liquid chromatography [56] after derivatization with o -phthaldialdehyde (OPA) [67] . Leaves were ground in liquid nitrogen and resuspended in methanol/chloroform/water (12:5:3, v/v). After incubation at room temperature for 24 h, the homogenate was centrifuged at 1,500 g for 30 min and the resulting supernatant mixed with chloroform/water (4:1:1.5, v/v/v). After decanting for 24 h, the aqueous phase was separated and subjected to derivatization by mixing with 50 mM OPA, 1% 2-mercaptoethanol in 400 mM borate buffer pH 9.5 (1:3, v/v) for 2 min. The OPA derivatives content were determined by reverse-phase HPLC (Shimadzu Corporation, Kyoto, Japan) using a Waters Spherisorb ODS2 C-18 column (4.6 μm, 4.6 × 250 mm) eluted at 0.8 ml min −1 by a linear gradient formed by solutions A (65% methanol) and B (50 mM sodium acetate, 50 mM disodium phosphate, 1.5 ml acetic acid, 20 ml tetrahydrofuran, 20 ml methanol in 1 l water, pH 7.2). The gradient increased the proportion of solution A from 20 to 60% between 0 and 25 min, 60 to 75% from 25 to 30 min and 75 to 100% from 30 to 50 min. The column effluent was monitored by a Shimadzu fluorescence detector (model RF-10AXL) operating at an excitation of 250 nm and emission of 480 nm. Amino acids were identified by their respective retention times and values compared with those of an amino acid standard solution (AA-S-18, Sigma Aldrich, plus 250 mM asparagine, glutamine and gamma-aminobutyric acid) and normalized by fresh weight of leaf tissue. Gene expression analysis For real-time PCR analysis, total RNA was extracted with Trizol (Invitrogen) and ethanol precipitation, and subsequently treated with Amplification Grade DNAse I (Invitrogen). The cDNA was synthesized using Im-Prom II reverse transcriptase (Promega, Fitchburg, WI), as recommended by the manufacturer. Gene expression analysis was carried out using Platinum SYBR Green qPCR Supermix-UDG (Invitrogen) in a Real-Time PCR System 7500 (Applied Biosystem, Foster City, CA). Gene expression was calculated with the 2 −ΔΔ C t method [68] with Actin2 as internal standard [69] . All gene-specific primers used in this study are shown in the Supplementary Table 1 . In vitro and in vivo S- nitrosylation assays Leaf extracts from 35S::FLAG-GSNOR1 in WT or nox1 plants were mock-treated or S -nitrosylated in vitro with 500 μM of Cys-NO for 20 min in the dark. Excess Cys-NO was removed using Zeba desalting columns (Thermo Fisher Scientific) and proteins subjected to the biotin switch technique as described previously [42] . Biotinylated proteins were pulled down with streptavidin agarose CL-6B (Thermo Fisher Scientific) and FLAG-GSNOR1 protein detected by western blotting with an anti-Flag M2 clone antibody (1:2,000 or 1:2,500, Sigma Aldrich, cat. no. F3165) ( Supplementary Fig. 8 ). How to cite this article: Frungillo, L. et al. S -nitrosothiols regulate nitric oxide production and storage in plants through the nitrogen assimilation pathway. Nat. Commun. 5:5401 doi: 10.1038/ncomms6401 (2014).